Photoactuators and motors based on carbon nanotubes with selective chirality distributions Direct conversion of light into mechanical work, known as the photomechanical effect, is an emerging field of research, largely driven by the development of novel molecular and polymeric material systems. However, the fundamental impediment is that the previously explored materials and structures do not simultaneously offer fast and wavelength-selective response, reversible actuation, low-cost fabrication and large deflection. Here, we demonstrate highly versatile photoactuators, oscillators and motors based on polymer/single-walled carbon nanotube bilayers that meet all the above requirements. By utilizing nanotubes with different chirality distributions, chromatic actuators that are responsive to selected wavelength ranges are achieved. The bilayer structures are further configured as smart ‘curtains’ and light-driven motors, demonstrating two examples of envisioned applications. Reconfigurable materials that change their shape and functionality in response to external stimuli represent a novel class of materials that enable new applications [1] , [2] , [3] , [4] , [5] , [6] , [7] . Previous work includes shape-reconfigurable structures based on shape memory polymers [8] , [9] , bimorphs [10] , [11] , molecular motors [12] , [13] , [14] and hydrogels [15] , [16] that respond to light or heat. For example, azobenzene functional materials have been utilized for photoactuators based on cis – trans transformation driven by light irradiation [12] , [17] , [18] . However, the need for dual wavelength operation (UV and visible) for reversible actuation and slow response time (~10 s) limit their practical utility for certain applications [12] , [17] , [18] . Recently, nanotube-based photoactuation has been reported using different platforms, including bilayers [19] , composites [20] and cantilever structures [21] , showing the promise of nanotubes for such applications. The principle actuation mechanism for most of these reported devices has been attributed to photo-induced charge build-up at the interfaces. Here, we present a simple photoactuator device concept based on single-walled carbon nanotube (SWNT)/polymer bilayers that takes advantage of the highly intriguing photothermal properties of SWNTs. The actuators deliver large deflection, fast (~0.5 s) and user-defined, wavelength-selective response. Previous studies have utilized the strong optical absorbance of SWNTs [22] in the near-infrared regime to induce significant local heating for photothermal cancer therapy. Furthermore, recent developments in the chirality purification of SWNTs have enabled the design of materials with desirable absorption properties and selective spectral response [23] , [24] , [25] . Building on these advancements, here we report a new class of highly versatile photoactuators based on SWNTs, with potential applications in smart curtains for energy-efficient windows, camouflage, sun-driven motors and oscillators, and monochromatic light sensors. 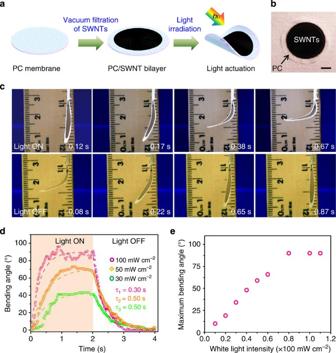Figure 1: PC/SWNT bilayer photoactuators. (a) Schematics illustrating the PC/SWNT bilayer structure. (b) Optical image of a circular PC/SWNT (10 μm/1 μm in thickness) bilayer with a diameter of 25 mm made by vacuum filtration (scale bar, 5 mm). (c) Series of optical images showing the light-actuation process of a bilayer structure with HiPCO nanotubes. The sample is held in air from the top edge, and illuminated with 100-mW cm−2white light normal to its surface (light is incident from the left side). The first and second row images correspond to the bending (light on) and unbending (light off) processes, respectively. (d) Bending angle as a function of time as light is turned on (time, 0 s) and off (time, 2 s) for different illumination intensities. The circle data points are from experiments, and the dashed lines represent the exponential fits. (e) Maximum (i.e., steady state) bending angle as a function of solar light intensity. Polymer/SWNT bilayers Figure 1a schematically illustrates the fabrication process of polymer/SWNT bilayers. The process is facile and scalable, which only involves vacuum filtration of a SWNT solution on a 10-μm-thick polycarbonate (PC) membrane (0.4 μm pore size). An optical image of a fabricated PC/SWNT bilayer structure is shown in Fig. 1b . The SWNTs form densely packed thin films on top of the PC membrane as seen from the scanning electron microscopy images in Supplementary Fig. S1 . The thickness of the SWNT thin-film is controlled from ~0.2 to 2 μm by adjusting the total amount of the filtered SWNTs ( Supplementary Fig. S2 ). Three types of nanotubes were explored: HiPCO, metal-enriched and (6,5) chirality-enriched SWNTs. In this bilayer structure, the SWNTs serve as an excellent light absorber layer with the specific wavelength range of absorption dependent on the type of nanotubes used [26] . The absorbed photon energy in nanotubes is readily converted to heat, which is then transported to the PC layer. The vacuum filtration ensures a mechanically coherent SWNTs/PC interface for effective heat transfer between the two layers. As the PC membrane has a large coefficient of thermal expansion of ~65 p.p.m. per Kelvin [27] , which is over 10 × larger than that of SWNTs (<4 p.p.m. per Kelvin) [28] , the structure is strongly curled (that is, deflected) towards the SWNT side upon light irradiation ( Fig. 1a , right panel). Figure 1: PC/SWNT bilayer photoactuators. ( a ) Schematics illustrating the PC/SWNT bilayer structure. ( b ) Optical image of a circular PC/SWNT (10 μm/1 μm in thickness) bilayer with a diameter of 25 mm made by vacuum filtration (scale bar, 5 mm). ( c ) Series of optical images showing the light-actuation process of a bilayer structure with HiPCO nanotubes. The sample is held in air from the top edge, and illuminated with 100-mW cm −2 white light normal to its surface (light is incident from the left side). The first and second row images correspond to the bending (light on) and unbending (light off) processes, respectively. ( d ) Bending angle as a function of time as light is turned on (time, 0 s) and off (time, 2 s) for different illumination intensities. The circle data points are from experiments, and the dashed lines represent the exponential fits. ( e ) Maximum (i.e., steady state) bending angle as a function of solar light intensity. Full size image Photoresponse of bilayer actuators The fast and reversible photoactuation of the PC/SWNT structures is evident from the optical photographs shown in Fig. 1c . Here, HiPCO nanotubes are used [29] . When the PC/SWNT bilayer is placed directly under a solar simulator with 1-sun intensity (100 mW cm −2 ), the sample is bent ~90° within ~0.67 s and reverts back to the relaxed (that is, flat) state in ~0.87 s after the light is turned on and off, respectively. By using a high-speed video camera (1,200 frames per second), the bending angle of the actuator is captured and plotted as a function of time for different illumination intensities ( Fig. 1d ). The bending and unbending processes can both be fitted with an exponential response using equations (1) and (2): where θ 0 is the maximum bending angle, t is time and τ is the actuation response time constant. The actuation response time constant is extracted to be ~0.50 s for both bending and unbending, which is significantly faster than the azobenzene-based polychromic materials with a response time of ~10 s [12] . The fast response is attributed to the low heat capacity [30] , high thermal conductivity ( Supplementary Fig. S3 ) [31] and the excellent near-infrared light absorption of the SWNT thin film [32] , making them ideal photothermal material. Owing to the superb optical absorbance properties of SWNTs, the PC/SWNT photothermal actuator is highly sensitive to light irradiation. Figure 1e exhibits the maximum bending angle as a function of the light intensity; an easily detectable bending angle of ~10° is found at 10 mW cm −2 (0.1 sun). The bending angle starts to saturate at ~90° when the illumination intensity is >80 mW cm −2 (0.8 sun). Interestingly, further increase of the intensity causes the structure to oscillate around its saturation bending angle (90°) due to the shadowing effect. Specifically, as the bending angle becomes slightly larger than 90°, part of the SWNT film becomes blocked from light irradiation due to self-shadowing, hence driving the oscillation process. This phenomenon is depicted in the Supplementary Movie 1 , where an oscillation frequency of ~5 Hz is observed for continuous 1.2-sun illumination. Photothermal actuation mechanism To elucidate the underlying photothermal mechanism of the PC/SWNT bilayers, we used an infrared camera to measure the real-time temperature change of the sample upon light irradiation (see Methods for details of the set-up). 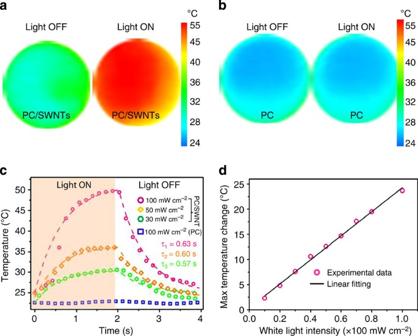Figure 2: Photothermal characterization of PC/SWNT bilayers. (a) Infrared images of a PC/SWNT bilayer with and without light illumination (100 mW cm−2, white light). (b) Infrared images of a blank PC film used as a control with and without light illumination (100 mW cm−2). (c) Temperature measurements of a PC/SWNT bilayer as light is turned on (time, 0 s) and off (time, 2 s) for different illumination intensities. (d) Maximum temperature rise of the PC/SWNT bilayer as a function of solar light intensities. For panelsa–dHiPCO nanotubes were used with a film thickness of 1 μm. Figure 2a shows the temperature profile of a PC/SWNT bilayer film (10 μm/1 μm) when the light is on and off. It is evident that the temperature of the substrate is increased by ~20 °C under 1-sun illumination. In contrast, no observable temperature change is found in the PC film without SWNTs ( Fig. 2b ). Figure 2c shows the temperature of a PC/SWNT bilayer as a function of exposure time to light with various illumination intensities. Rapid temperature rise and decay are clearly observed. A thermal time constant (corresponding to 63% drop in temperature) of ~0.60 s is extracted similar to Fig. 1d . This extracted thermal time constant is close to the actuation response time constant ( Fig. 1d ), which confirms the underlying photothermal actuation mechanism. As shown in Fig. 2d , the maximum temperature change and light intensity show near-linear dependency. The comparison between Figs 1e and 2d indicates that a 5°C change in the temperature (corresponding to 20 mW cm −2 illumination) results in a bending angle of ~20°, depicting the high sensitivity of the system. The photothermal effect of PC/SWNT bilayers with various SWNT layer thicknesses was also investigated and summarized in Supplementary Table S1 . We also carried out control experiments inside an oven to induce pure thermal actuation. The bending angle measurements from these control experiments are consistent with the photoactuation experiments for the same temperature change as shown in Supplementary Fig. S4 and Supplementary Table S2 . Figure 2: Photothermal characterization of PC/SWNT bilayers. ( a ) Infrared images of a PC/SWNT bilayer with and without light illumination (100 mW cm −2 , white light). ( b ) Infrared images of a blank PC film used as a control with and without light illumination (100 mW cm −2 ). ( c ) Temperature measurements of a PC/SWNT bilayer as light is turned on (time, 0 s) and off (time, 2 s) for different illumination intensities. ( d ) Maximum temperature rise of the PC/SWNT bilayer as a function of solar light intensities. For panels a – d HiPCO nanotubes were used with a film thickness of 1 μm. Full size image Next, we focus on understanding the time-limiting step in the actuation of our bilayers by calculating the thermal time constant of both SWNT and PC films ( Supplementary Note 1 ). First, we estimated the average heat transfer coefficient of free air convection of the two surfaces of PC/SWNT from the equilibrium temperature change under solar light irradiation according to the following equation: 2 h Δ T = W in . Here, h is the average heat transfer coefficient, Δ T is the equilibrium temperature change and W in is the power density of solar irradiation. The estimated heat transfer coefficient is 20.6 W m −2 K −1 . The thermal time constant is then calculated according to τ = ρCb / h , where ρ is mass density of the film; C is the specific heat; b is the thickness of the film. The calculated thermal time constants of the SWNT and PC films are 0.04 and 0.7 s, respectively. Clearly, the heat capacity in the PC layer dominates the response time with the calculated value matching the experiments well, suggesting that the proposed operation mechanism is indeed viable ( Fig. 2c ). Mechanical modelling Mechanical modelling was performed to quantitatively study the effect of SWNT film thickness and the maximum temperature change on the static maximum bending angle ( Fig. 3 ). The sample receives non-uniform illumination due to mechanical curling of the actuator ( Fig. 3a ). Based on the bimetal thermostat equation of Timoshenko [33] , we developed an analytical model for the bending angle with non-uniform light irradiation ( Supplementary Note 2 ). From modelling, the effect of SWNT film thickness (PC thickness of 10 μm) on the maximum bending angle for a given illumination intensity is calculated. The modelling matches the experimental results well ( Fig. 3b ). The maximum deflection increases with SWNT film thickness up to ~1 μm, beyond which further increase in the SWNT thickness has minimal effect. The results show that a high degree of control in the dynamic range of our bilayer actuators can be obtained by simply tuning the thickness of the SWNT film as compared with that of the PC substrate. The conversion efficiency of our actuators (defined as the generated elastic energy due to photoactuation divided by the incident light energy) is estimated to be ~0.01% ( Supplementary Note 3 ). It is noted that this energy conversion efficiency is for doing internal work on deforming the bilayer rather than for doing external work. 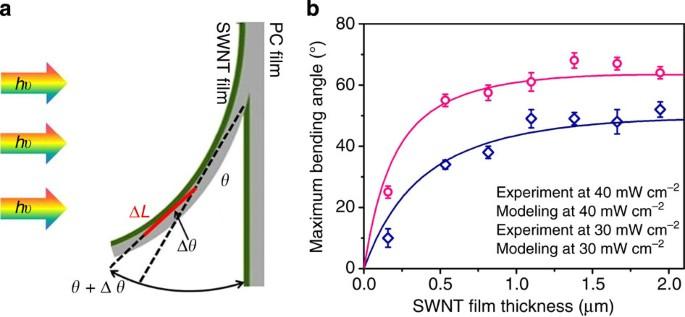Figure 3: Mechanical modelling of PC/SWNT actuators. (a) A bilayer model used in the mechanical simulation. Because of the difference in coefficient of thermal expansion, a bilayer PC/SWNT structure with a lengthLis deflected to a curvature radius ofRand bending angle ofθwhen heated by light illumination. Here, the edge of the structure is fixed in position, similar to those of the actuator experiments. (b) Modelling and experimental results for the maximum bending angle as a function of SWNT film thickness. The thickness of the PC layer is fixed at 10 μm. Figure 3: Mechanical modelling of PC/SWNT actuators. ( a ) A bilayer model used in the mechanical simulation. Because of the difference in coefficient of thermal expansion, a bilayer PC/SWNT structure with a length L is deflected to a curvature radius of R and bending angle of θ when heated by light illumination. Here, the edge of the structure is fixed in position, similar to those of the actuator experiments. ( b ) Modelling and experimental results for the maximum bending angle as a function of SWNT film thickness. The thickness of the PC layer is fixed at 10 μm. Full size image User-defined, wavelength-selective response A unique feature of the PC/SWNT photothermal actuators is the tunability of the responsive wavelength range by using nanotubes with different chirality distributions. It is known that the light absorption characteristics of carbon nanotubes are determined by their chiralities [26] . To demonstrate this feature, in addition to using as-synthesized HiPCO tubes with a mixture of chiralities, we used 98% purity metallic nanotubes (as-received from NanoIntegris) with M 11 absorption peak at ~700 nm (average nanotube diameter of 1.4 nm), and (6,5) single-chirality nanotubes prepared as previously described [24] (purity>97%) with S 22 and S 11 absorption peaks at ~560 nm and 970 nm, respectively ( Fig. 4a,b ). For the light-actuation experiments, three illumination wavelength bands of 600–800 nm, 850–1,050 nm and 1,050–1,250 nm were created by using a combination of long- and short-pass optical filters. The power of the light source was calibrated to maintain the same transmitted power for all three wavelength bands. As expected, HiPCO nanotubes are responsive to all three wavelength bands ( Fig. 4c ). In contrast, the actuators with metal-enriched nanotubes are only responsive to the visible wavelength band of 600~800 nm. On the other hand, actuators with single-chirality (6,5) nanotubes only respond to the 850–1,050 nm band. The wavelength-dependent response is also evident from the photothermal measurements ( Supplementary Fig. S5 ). This feature represents a useful and unique aspect of the actuators that takes advantage of the intriguing optical properties of nanotubes. 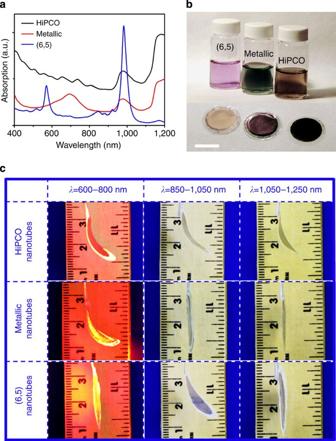Figure 4: Chromatic photoactuators made from nanotubes with different chirality distributions. (a) Optical absorption spectra for HiPCO, metallic and (6,5)-enriched nanotube films. (b) Optical image of the bilayer structures made from HiPCO, metallic, and single-chirality-enriched nanotubes along with their corresponding nanotube solutions (scale bar, 15 mm). (c) Light response of the three different bilayers from panelbfor wavelength bands of 600–800 nm, 850–1,050 nm and 1,050–1,250 nm. For each wavelength band, the power is calibrated to maintain the same transmitted power of ~35 mW cm−2. Light is incident from the right side of the image, normal to the surface of the samples. Figure 4: Chromatic photoactuators made from nanotubes with different chirality distributions. ( a ) Optical absorption spectra for HiPCO, metallic and (6,5)-enriched nanotube films. ( b ) Optical image of the bilayer structures made from HiPCO, metallic, and single-chirality-enriched nanotubes along with their corresponding nanotube solutions (scale bar, 15 mm). ( c ) Light response of the three different bilayers from panel b for wavelength bands of 600–800 nm, 850–1,050 nm and 1,050–1,250 nm. For each wavelength band, the power is calibrated to maintain the same transmitted power of ~35 mW cm −2 . Light is incident from the right side of the image, normal to the surface of the samples. Full size image Smart curtains Finally, we focus on the use of PC/SWNT actuators for practical applications. In one example, we demonstrate their use for ‘smart’ curtains that can be engineered to be either closed or opened upon sunlight illumination ( Fig. 5 ). Here, circular PC/SWNT bilayers are mounted on a surface by their top edge only. Two types of bilayers based on HiPCO nanotubes are utilized ( Fig. 5a ). One involving the configuration discussed above, which curls up (that is, opens) on light illumination (Type A). The other operates in the reverse mode—that is being curled open in the absence of light and closing (that is, moving to the flat state) on light illumination (Type B). To fabricate Type B actuators, PC/SWNT bilayers are pre-strained at 70 °C for 12 h to make them curled to the PC side. By arraying the circular actuators on a stage with each actuator being mounted by the top edge, a curtain is obtained that either closes (Type B) or opens (Type A) by light illumination ( Fig. 5b,c , and Supplementary Movie 2 ). Besides energy-efficient windows, this smart curtain may be potentially useful for camouflage applications. 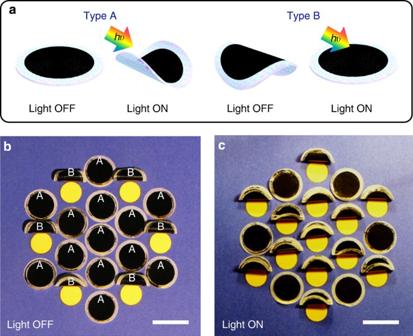Figure 5: Smart curtains. (a) Schematic for two different types of PC/SWNT photoactuators made by tuning the built-in strain of the bilayers. Type A is flat (that is, closed) in the absence of sunlight and is curled (that is, open) when exposed to sunlight. Type B is reversed (that is, open in the absence of light and closed under light). (b,c) Hexagonal array of 19 bilayer actuators (13 Type A and 6 Type B) when simulated sunlight is off and on, respectively. The circular actuators are mounted on a blue cardboard by their top edge only. The region underneath the actuators is marked yellow, so that when the actuators are open, the effect is clearly visible. Here, HiPCO nanotubes were used (scale bar, 25 mm). Figure 5: Smart curtains. ( a ) Schematic for two different types of PC/SWNT photoactuators made by tuning the built-in strain of the bilayers. Type A is flat (that is, closed) in the absence of sunlight and is curled (that is, open) when exposed to sunlight. Type B is reversed (that is, open in the absence of light and closed under light). ( b , c ) Hexagonal array of 19 bilayer actuators (13 Type A and 6 Type B) when simulated sunlight is off and on, respectively. The circular actuators are mounted on a blue cardboard by their top edge only. The region underneath the actuators is marked yellow, so that when the actuators are open, the effect is clearly visible. Here, HiPCO nanotubes were used (scale bar, 25 mm). Full size image Motors and oscillators As a second application demonstration of PC/SWNT actuators, we have fabricated a 2-cm-sized motor, which rolls away from the direction of light illumination. The motor is fabricated by assembling three pieces of rectangular (2 cm × 2.5 cm) PC/SWNT (25 μm/1 μm) film together into a cylinder with the SWNT side facing outwards. As illustrated in Fig. 6a,b , non-uniform illumination on the motor from an angled light source causes the curvature to decrease on the light-facing side, that is, the location that gets more illumination has the tendency to be flattened. This causes a change to the centre of mass of the motor, thereby resulting in a torque that drives the motor away from light on a flat surface at a speed of ~6 cm s −1 ( Fig. 6c and Supplementary Movie 3 ). On the other hand, an oscillating wheel is made by making a roller with elliptical cross-section. In this case, the structure leans forward and backward at a frequency of ~2 Hz on light illumination ( Supplementary Movie 4 ). These demonstrations illustrate macro-scale motors with fast mechanical motion driven by a single light source, which can only be realized with fast and reversible light-responsive materials. As cyclic lifetime is critically important for practical use, we have measured 60,000 cycles of actuation test on a PC/SWNT bilayer. The deformation remains unchanged as shown in Supplementary Fig. S6 and Supplementary Movie 5 . 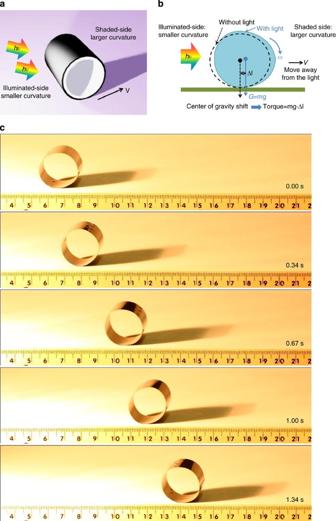Figure 6: A fast forward-moving motor driven by light. (a) Schematic showing the operation scheme of the motor under light. The motor consists of a PC/SWNT bilayer (25 μm/1 μm in thickness) that is rolled into a tubular structure (diameter of ~2 cm; length of ~2.5 cm). (b) Schematic showing the displacement in the center of gravity of the motor due to the directional light exposure. The induced torque drives the motor away from the light source. (c) Optical image series as a function of time showing a forward-moving motor driven by a halogen lamp. Figure 6: A fast forward-moving motor driven by light. ( a ) Schematic showing the operation scheme of the motor under light. The motor consists of a PC/SWNT bilayer (25 μm/1 μm in thickness) that is rolled into a tubular structure (diameter of ~2 cm; length of ~2.5 cm). ( b ) Schematic showing the displacement in the center of gravity of the motor due to the directional light exposure. The induced torque drives the motor away from the light source. ( c ) Optical image series as a function of time showing a forward-moving motor driven by a halogen lamp. Full size image In summary, PC/SWNT bilayer photoactuators with highly unique light-responsive properties were fabricated using a facile and low-cost room-temperature process. The PC/SWNT bilayers simultaneously offer fast response, extreme light sensitivity, large deflection and reversible actuation. By using SWNTs with different chirality distributions, the responsive wavelength range of the actuators is readily programmed, enabling the development of chromic actuators. As a benchmark for fast and reversible light-responsive properties, a smart curtain and a fast-moving motor have been demonstrated to highlight two representative applications of the proposed bilayers. Moving forward, the bilayer actuators can be optimized in terms of SWNT and polymer thickness, and polymer Young’s modulus to achieve larger force output, depending on the application needs. By exploiting nanotube-printing strategies on polymer substrates, this work can be extended in the future to the fabrication of complex, reconfigurable structures using a scalable process scheme. PC/SWNT bilayer fabrication Purified HiPCO SWNT powder is purchased from NanoIntegris Inc. (residual Fe catalyst <15 wt%, diameter 0.8–1.2 nm, length 100–1,000 nm). A 0.5-mg ml −1 aqueous solution of SWNTs is made using 2% sodium deoxycholate as surfactant. After 400 min of sonication (Crest Ultrasonics 275DA; power 9), large SWNT aggregates, non-SWNT carbonaceous impurities, and metal catalyst particles were removed by centrifuging the SWNT dispersion for 10 min with 13,000 g rotation speed. Vacuum filtration is performed using a standard 25-mm set up with a PC membrane (Millipore, 0.4-μm pore size, 25 mm diameter). After filtration, 20 ml water is added to rinse away the surfactant. A similar fabrication process is used to obtain actuators with metallic and (6,5)-enriched nanotubes (with a concentration of ~0.01 mg ml −1 ). All three actuators have the same SWNT film thickness of ~1 μm by controlling the amount of SWNTs used for the filtration. Temperature measurements of the PC/SWNT bilayers For the infrared camera measurements, the entire edge of the sample is fixed onto a piece of cardboard with a 20-mm hole so that the sample is mostly suspended in air and thermally well insulated. The temperature of the SWNT film surface is measured by an infrared camera. The camera is 25 mm away from the sample with 30° detection angle with respect to the surface normal of the sample. How to cite this article: Zhang, X. et al . Photoactuators and motors based on carbon nanotubes with selective chirality distributions. Nat. Commun. 5:2983 doi: 10.1038/ncomms3983 (2014).